Relativistic electron mirrors from nanoscale foils for coherent frequency upshift to the extreme ultraviolet Reflecting light from a mirror moving close to the speed of light has been envisioned as a route towards producing bright X-ray pulses since Einstein’s seminal work on special relativity. For an ideal relativistic mirror, the peak power of the reflected radiation can substantially exceed that of the incident radiation due to the increase in photon energy and accompanying temporal compression. Here we demonstrate for the first time that dense relativistic electron mirrors can be created from the interaction of a high-intensity laser pulse with a freestanding, nanometre-scale thin foil. The mirror structures are shown to shift the frequency of a counter-propagating laser pulse coherently from the infrared to the extreme ultraviolet with an efficiency >10 4 times higher than in the case of incoherent scattering. Our results elucidate the reflection process of laser-generated electron mirrors and give clear guidance for future developments of a relativistic mirror structure. The properties of an electromagnetic wave reflected off a mirror moving with a velocity β = v/c towards the observer are indeed intriguing; in the classical picture, the frequency and amplitude of the reflected wave are enhanced by a factor 4 γ 2 , where γ =(1− β 2 ) −1/2 , whereas the reflected pulse is compressed in time by 1/4 γ 2 , resulting in an ultimate increase in peak brightness for the reflection of an electromagnetic wave off an ideal relativistic mirror [1] . For example, if a mirror with a γ =10 could be produced, a laser with a duration of 10 fs and wavelength of 800 nm would be upshifted to a wavelength of 2 nm and compressed to a pulse duration of 25 as. The creation of a relativistic structure, which acts as an efficient mirror in the short wavelength range is demanding. An energetically feasible approach is to use relativistic electrons to reflect laser photons via Thomson scattering. Although conventional accelerators can reach very high electron energies γmc 2 and are an effective tool for upshifting optical laser photons to X-ray energies [2] , they do not form a reflecting structure analogous to a mirror because of their long bunch duration, and therefore the Thomson-scattered radiation is incoherent. In contrast, coherent, mirror-like reflection can be obtained from dense electron sheets, where the thickness of the sheet is small compared with the wavelength of the reflected radiation in the rest frame of the electron sheet. The advent of ultra-high-intensity lasers allows reflecting structures consisting of relativistic electron sheets to be produced, which satisfy these conditions. Different schemes have been developed to create such relativistic structures in plasmas on a microscale. In particular, high harmonic generation via the reflection off a relativistically oscillating plasma surface has raised great interest [3] , owing to its capacity to create short bursts of radiation in the extreme ultraviolet (XUV). However, this process intrinsically produces radiation in a wide spectral range [4] , [5] . Achieving a controlled, narrow-band frequency shift, which allows to entirely frequency-convert the counter-propagating laser to high frequencies, as envisaged in the ideal picture, requires generating a reflective structure propagating with a constant velocity. Such structures can indeed be produced in a laser-driven plasma wake wave in low-density plasmas formed by the interaction of the laser with a gaseous target [6] , [7] . The limitation of this approach is that the γ -factor of the plasma density wake is determined by the group velocity of the laser and, thus, requires decreasing density (and hence reflectivity) to achieve large γ -factors. We therefore turn our attention to solid targets, which have substantially higher initial density. The generation of solid density, relativistic electron mirrors (REMs) from nanometre-scale thin foils has recently been investigated theoretically. In the limit of laser pulses with extremely fast rise time, all the electrons in a nanofoil can be expelled in a single, dense sheet, propagating at relativistic velocities [8] . Although ultimately limited by Coulomb explosion, the electron sheet was shown to be stable over micrometre-scale distances [9] , sufficiently long for the coherent backscattering of a probe pulse. Under the correct conditions [10] , the laser frequency ω L can be upshifted to a narrow band of frequencies centred around 4γ 2 ω L —thereby acting like the relativistic mirror first described by Einstein. To ‘blow out’ all the foil electrons, the ponderomotive force F p ( v / c ) × B L ~ E L must overcome the electrostatic field binding the electrons to the ions in the foil E s =4 πen 0 l 0 . This allows the required intensity of the laser [μm] 2 to be estimated as a 0 >2 π ( l 0 / λ L )( n 0 / n c ), where a 0 = eE L / mcω L is the normalized vector potential, is the critical plasma density, n 0 and l 0 are the foil density and thickness, and E L is the laser field, respectively. For diamond-like carbon foils with densities of 470 n c and l 0 =5 nm reaching the blow-out condition corresponds to intensities of >10 21 W cm −2 in a pulse with single-cycle rise time. Although these conditions are still somewhat beyond what can be achieved experimentally, existing lasers are fast approaching such parameters [11] and lasers that should reach ‘blow-out’ conditions are currently being built. Here we investigate the generation of REMs from nanometre foils using current state-of-the-art high-intensity laser pulses with slightly longer pulses (tens of femtoseconds). A detailed numerical study shows that dense, relativistic electron sheets can already be created from the interaction of an intense (50 fs) pulse with a nanoscale foil. We demonstrate the coherent backscattering from those REMs in a dual beam experiment observing a relativistic Doppler shift from 800 nm down to ~60 nm. Computer simulation To elucidate the detailed dynamics of such an interaction, we conduct particle-in-cell (PIC) simulations with realistic laser-pulse parameters, that is, 6 × 10 20 W cm −2 , 50 fs in combination with a 10-nm thin, fully ionized carbon foil and a weak (6 × 10 15 W cm −2 ) probe pulse interacting with the back of the foil. The main driving term generating the mirror structure is the ponderomotive force (radiation pressure) of the incident laser pulse, acting on the skin layer of the solid plasma at a frequency of 2 ω L . As a result, dense electron bunches are formed at the boundary and accelerated into the plasma via the Lorentz force, periodically, at every half cycle of the laser field [12] , [13] , [14] . Each of these bunches traverses the thin plasma within much less than a femtosecond, and escapes into the vacuum region at the rear side of the plasma as a nanometre-thin, relativistic electron sheet, with density up to a few percent of solid (as shown in Fig. 1a ) and a velocity component along the laser axis β z . 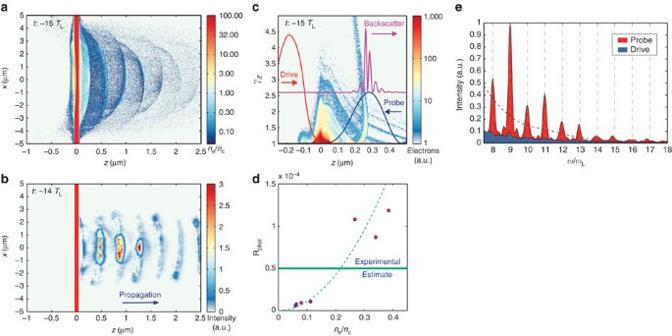Figure 1: Reflection from relativistic electron mirrors. (a) Electron densityne(in units ofnc, logarithmic scale) showing the periodic emission of dense electron bunches at every half cycle of the driving laser field. (b) Frequency-filtered probe field intensity (filter:ω/ωL>5). The counter-propagating probe pulse (not shown here) reflects off the created relativistic electron mirrors, causing the periodic emission of intense, attosecond short radiation. (c) Lineout of the electron mirrorγ-factorγz=(1−βz2)−1/2versusz(averaged in transverse dimension within ±1 μm aroundx=0 μm, logarithmic scale) superimposed with the normalized intensity lineout of the incident and reflected pulses. The mirror structure is sharply located in space, reflects off the probe pulse in the vacuum region behind the target and causes a frequency upshift governed by (1+βz)2γz2ωL. (d) Reflectivity of the generated electron mirrors analysed for a backreflected wavelength of 80 nm (band width: 20%) as a function of the number of electrons involved in the reflection process, that is all electrons within the mirror structure with (1+βz)2γz2=10 (band width: 20%). The reflectivity obtained from PIC simulation (dots) follows a quadratic scaling, as expected from coherent scattering theory (analytic curve). The best estimate of the experimentally observed reflectivity is 5 × 10−5(green line), in fair agreement with the expected value. The estimate for the electron mirror reflectivity is discussed in detail in the Methods section. (e) Spectrum of the drive and probe field recorded behind the target normalized to the continuous background level. Dashed curve: spectrum (rescaled) of one isolated backscattered pulse. Figure 1: Reflection from relativistic electron mirrors. ( a ) Electron density n e (in units of n c , logarithmic scale) showing the periodic emission of dense electron bunches at every half cycle of the driving laser field. ( b ) Frequency-filtered probe field intensity (filter: ω / ω L >5). The counter-propagating probe pulse (not shown here) reflects off the created relativistic electron mirrors, causing the periodic emission of intense, attosecond short radiation. ( c ) Lineout of the electron mirror γ -factor γ z =(1− β z 2 ) −1/2 versus z (averaged in transverse dimension within ±1 μm around x =0 μm, logarithmic scale) superimposed with the normalized intensity lineout of the incident and reflected pulses. The mirror structure is sharply located in space, reflects off the probe pulse in the vacuum region behind the target and causes a frequency upshift governed by (1+ β z ) 2 γ z 2 ω L . ( d ) Reflectivity of the generated electron mirrors analysed for a backreflected wavelength of 80 nm (band width: 20%) as a function of the number of electrons involved in the reflection process, that is all electrons within the mirror structure with (1+ β z ) 2 γ z 2 =10 (band width: 20%). The reflectivity obtained from PIC simulation (dots) follows a quadratic scaling, as expected from coherent scattering theory (analytic curve). The best estimate of the experimentally observed reflectivity is 5 × 10 −5 (green line), in fair agreement with the expected value. The estimate for the electron mirror reflectivity is discussed in detail in the Methods section. ( e ) Spectrum of the drive and probe field recorded behind the target normalized to the continuous background level. Dashed curve: spectrum (rescaled) of one isolated backscattered pulse. Full size image The ejected electron bunches thus fulfil the condition for coherent scattering of counter-propagating light and form a series of partially reflective REMs. In counter-propagating geometry, the scattering amplitudes of the backscattered radiation add up constructively in direction normal to the mirror surface [15] and the mirror acts in the way one would expect intuitively, that is, the radiation is reflected in the specular direction ( Fig. 1b ). Note that the REM is formed by electrons, which are not propagating exactly at the same direction or at the same velocity. However, the velocity dispersion is sufficiently small for the REM to remain intact over micron-scale distances—sufficient for coherent reflection to take place. The REM can be described by an effective γ -factor [15] , [16] determined by the velocity component of the mirror in its normal direction β z , thus γ z =(1− β z 2 ) −1/2 . As each mirror consists of electrons of various energies ( Fig. 1c ), the backscattered radiation is shifted to a continuous spectrum, giving rise to coherent spectral contributions up to a frequency of ω =(1+ β z ,max ) 2 γ z ,max 2 ω L from each of these mirrors. A clear signature of the coherent, mirror-like behaviour of the REM is the quadratic scaling of the emitted radiation on the number of electrons involved in a single reflection, as shown in Fig. 1d . The periodic REM formation results in a train of backscattered pulses ( Fig. 1b ). In the frequency domain, the emission of a train of backscattered pulses leads to spectral interference and, thus, a strongly modulated photon spectrum is expected. Subsequent REMs are ejected in opposite transverse direction due the alternating electric field of the driving laser and, hence, the temporal spacing of REMs emitted in similar direction is Δ T = T L , giving rise to spectral modulations at Δ ω =2 π /Δ T = ω L , as observed in the time-integrated frequency spectrum ( Fig. 1e ). Note that each of the mirrors is partially reflective for our experimental parameters, although the density of each mirror in the lab-frame is above the critical density of n c =1.1 × 10 21 / λ L [μm] 2 cm −3 at which a stationary plasma would become opaque to the probe wavelength of 800 nm. However, transforming in the rest frame of the mirror the wavelength of the probe is shifted to λ L ′= λ L /(1+ β z ) γ z and the effective mirror density is reduced to n e ′= n e / γ z . Thus, for our conditions each REM is expected to be partially reflective, as seen in Fig. 1c . Experimental results The experiments were conducted at the Astra Gemini Laser Facility–one of the most powerful lasers currently available. Nanometre-thin, freestanding foils were irradiated with a high-intensity ‘drive’ pulse at ultra-relativistic intensities (6 × 10 20 W cm −2 ), whereas a weaker, counter-propagating ‘probe’ pulse was focused to 10 15 W cm −2 —sufficiently weak so as not to perturb the interaction dynamics ( Fig. 2 ). 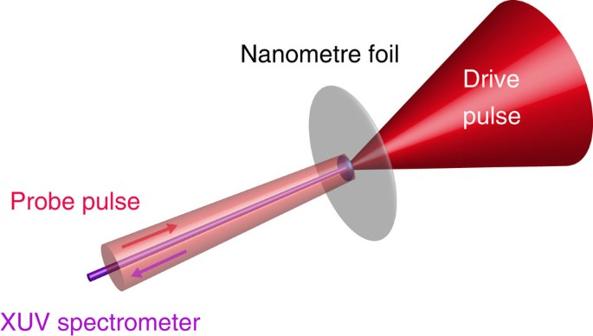Figure 2: Experimental set-up. The drive pulse (~5 J, 55 fs) is focused with an f/2 off-axis parabolic mirror to a focal spot of 3.5 μm full width at half maximum (FWHM) reaching peak intensities of 6 × 1020W cm−2. Simultaneously, the probe pulse (~2 mJ, 55 fs) is shot from the opposite side quasi counter-propagating (angle between both beam axis ~1°), focused with a lens (f/50) to a 55 μm FWHM spot corresponding to a peak intensity of 1 × 1015W cm−2. The radiation emitted from the foil is diagnosed at 0° with respect to target normal direction using a transmission grating spectrometer. Figure 2: Experimental set-up. The drive pulse (~5 J, 55 fs) is focused with an f/2 off-axis parabolic mirror to a focal spot of 3.5 μm full width at half maximum (FWHM) reaching peak intensities of 6 × 10 20 W cm −2 . Simultaneously, the probe pulse (~2 mJ, 55 fs) is shot from the opposite side quasi counter-propagating (angle between both beam axis ~1°), focused with a lens (f/50) to a 55 μm FWHM spot corresponding to a peak intensity of 1 × 10 15 W cm −2 . The radiation emitted from the foil is diagnosed at 0° with respect to target normal direction using a transmission grating spectrometer. Full size image The radiation observed with the XUV spectrometer shows no notable signal above noise level when irradiating 10- and 50-nm thin foils with the drive pulse only, Fig. 3a . The low-level modulation in the spectral intensity varies stochastically in consecutive shots. This behaviour changes when irradiating the target with the probe beam synchronously (see Fig. 3c ). Here a periodically modulated spectrum ranging down to ~60 nm wavelength is observed in good agreement with the PIC simulation, Fig. 1e , showing the periodic emission of REMs propagating with γ z ,max ~2 along the axis of the probe pulse, Fig. 1c . Such REMs scatter incident radiation coherently up to a frequency of ω =(1+ β z ,max ) 2 γ z ,max 2 ω L ~14 ω L . The spectral modulation due to the generation of multiple pulses is clearly visible and is in reasonable agreement with the spectrum obtained from PIC simulation. 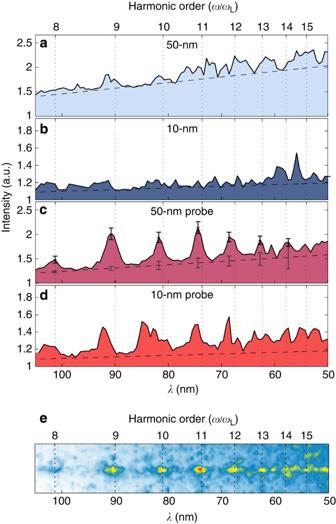Figure 3: Experimental spectra. Quantitative comparison of the measured XUV spectra obtained from a 50- and 10-nm foil irradiated with (a,b) the drive pulse only and (c,d) drive and probe pulses synchronously. The backscattered XUV radiation reveals a periodically modulated spectrum when irradiating the nanometre foils with the counter-propagating pulse, whereas the signal without the probe is shot noise-dominated. Ina–ddashed lines give the linear fit to the background. Inc, error bars on the fit line are the maximal deviation of the background noise from the linear fit, whereas error bars at the spectral peaks are signal noise deduced from photon counting statistics. The spectra shown here are representative for a data set comprising 25 target shots, both in single- and dual-pulse configuration. No signal was observed when irradiating the foil with the probe pulse exclusively (not shown here). (e) Detector image (hot pixels removed) obtained from a 50-nm probe shot. Figure 3: Experimental spectra. Quantitative comparison of the measured XUV spectra obtained from a 50- and 10-nm foil irradiated with ( a , b ) the drive pulse only and ( c , d ) drive and probe pulses synchronously. The backscattered XUV radiation reveals a periodically modulated spectrum when irradiating the nanometre foils with the counter-propagating pulse, whereas the signal without the probe is shot noise-dominated. In a – d dashed lines give the linear fit to the background. In c , error bars on the fit line are the maximal deviation of the background noise from the linear fit, whereas error bars at the spectral peaks are signal noise deduced from photon counting statistics. The spectra shown here are representative for a data set comprising 25 target shots, both in single- and dual-pulse configuration. No signal was observed when irradiating the foil with the probe pulse exclusively (not shown here). ( e ) Detector image (hot pixels removed) obtained from a 50-nm probe shot. Full size image In the simulations, the formation of the electron-density spikes is only observed for targets that are still opaque to the driving laser pulse close when the laser reaches its peak intensity. For our contrast conditions, 5-nm thin foils are marginal in this respect and, indeed, we observe no backscattered signal when irradiating 5-nm thin foils. On the other hand, the REMs quickly diminish in density and sharpness due to propagation, thus increasing the target thickness considerably hinders the formation of dense REMs behind the foil, while eventually favouring the emission of coherent synchrotron radiation [17] . The reflectivity (in terms of photon number) is estimated ~5 × 10 −5 at a backscattered wavelength of 80 nm (see Methods), in good agreement with the reflectivity observed in the PIC simulation shown in Fig. 1d . For comparison, the efficiency that would be expected for incoherent Thomson scattering is ~10 −9 , corresponding to a signal well below detection threshold in our experimental configuration. The generation of a laser like X-ray pulse via the reflection off a moving mirror is fascinating by its simplicity, and seemingly poses no restriction on the light pulse, which could be generated. In practice, the central aspect is the generation of a structure with high reflectivity, which we have demonstrated here for the first time experimentally for the XUV range. The generation of a mirror-like structure becomes increasingly challenging for shorter wavelengths. However, reaching higher γ -factors while maintaining high densities promises an intensity enhancement that scales as (1+ β z ) 4 γ z 4 , making the short-wavelength generation via reflection extremely beneficial. Accessing γ -factors of >10 and shifting the reflected radiation to the range of a few nanometres or even into the kiloelectronvolt range will require drive laser pulses that reach a 0 ~10–50 within one to two optical cycles, and has been shown to be possible in principle [16] , [18] . Achieving such performance would indeed be an exciting prospect. Ultra-thin foils 10-nm diamond-like carbon foils and 50-nm thin carbon foils were used in the experiment. The density of the target material was ~2.7 g cm −3 (diamond-like carbon) and ~2.1 g cm −3 (carbon), respectively. Laser-pulse contrast Nanometre-thin foils require high laser-pulse contrast to ensure the integrity of the foil at the arrival of the main pulse. To meet those high demands, a recollimating, double plasma mirror was introduced into the optical beam path of the drive laser, which improved the intrinsic contrast ratio of the laser system to 10 −9 measured at 2 ps before the arrival of the peak of the pulse using a third-order autocorrelator. Spatiotemporal overlap The foci of drive and probe pulse were accurately overlapped in space using high magnification imaging. The relative timing between both counter-propagating pulses was adapted by timing each pulse relative to a transverse probe pulse, using plasma shadowgraphy techniques. XUV spectrometer To characterize the XUV radiation a transmission, grating spectrometer was positioned along the target normal direction 1.3 m away from the target. The entrance of the spectrometer was defined by a pinhole with a 200-μm diameter, resulting in a detection angle of 1.7 × 10 −8 sr. The transmission grating with 1,000 lines per mm consists of freestanding gold wires supported by a triangular mesh structure. The XUV radiation was detected with a micro-channel plate that was imaged on a low-noise charge-coupled device camera. Particle-in-cell simulations Two-dimensional PIC simulations were performed using the PSC code [19] . The simulation parameters were matched close to the experimental conditions. Drive pulse: 6 × 10 20 W cm −2 , 50 fs pulse duration, 3 μm full width at half maximum focal spot, Gaussian pulse shape in space and time. Probe pulse: 6 × 10 15 W cm −2 , 100 fs pulse duration, 55 μm FHWM focal spot, Gaussian pulse shape in space, flattop in time. Both pulses were initialized in cross-polarized configuration. To account for a target pre-expansion due to limited laser contrast, the foil was modelled with 100-nm thickness and 47 n c density. The simulation box was 10 μm × 20 μm in longitudinal and transverse dimension, divided into 4,000 × 4,000 cells, using 200 particles per cell. A detector was positioned at z =3 μm in the simulation box to record the electric-field components of the drive and probe pulse behind the target during the interaction. Photon yield A rough estimate on the photon number can be given assuming a diffraction-limited light cone with apex angle given by the source size. We estimate 8 × 10 6 photons per shot at a wavelength of 80 nm within a band width of 20% and a solid angle of 7 × 10 −4 sr. This photon number should be viewed in context of the rather low probe intensity of 1 × 10 15 W cm −2 obtained in a loose focus of 55 μm full width at half maximum diameter. The size of our mirror is defined by the central region of the drive laser focus, ~2 μm ( Fig. 1b ). Moreover, the lifetime of the mirror is of the order of half an optical cycle. Accordingly, we estimate that 1.6 × 10 11 probe photons with 0.8-μm wavelength interact with the mirror and are reflected with an efficiency of ~5 × 10 −5 . The lower (upper) bound of the reflectivity estimate is 2 × 10 −5 (2 × 10 −4 ). Note that this photon reflectivity corresponds to an energy ratio of E 80 nm / E probe ~5 × 10 −4 due to the frequency upshift. The photon number could be increased substantially by increasing the probe intensity by ~10 3 up to the threshold of non-linear coherent Thomson scattering [18] . Moving to shorter, better contrast pulses has the potential to increase the REM density by ~10 2 to close to solid, which would correspond to an efficiency that is ~10 4 times greater for the wavelengths under consideration. As in our experimental configuration, the energy ratio of probe and drive pulse interacting with a mirror is ~1.6 × 10 −6 only, the efficiency with respect to the drive pulse is E 80 nm / E drive ~8 × 10 −10 , which can be enhanced by orders of magnitude based on the arguments above. Electron mirror reflectivity To deduce the reflectivity from the particle-in-cell simulation at a certain wavelength, we apply a spectral filter to the electron distribution of the acting mirror and the electric field of the backscattered radiation. The electric field is frequency-filtered within 9 ω L < ω <11 ω L and the peak intensity of the backscattered pulse is obtained from the resulting intensity distribution. The electron density of the corresponding electron bunch is filtered in phase space, such that all electrons satisfy 9<(1+ β z ) 2 γ z 2 <11 and the peak density of the remaining ‘monochromatic’ mirror is extracted. The ratio of incident and reflected intensity as observed in PIC simulation relates to the mirror reflectivity as from which we calculate the mirror reflectivity R m . As the electron-bunch density increases as the incident laser field rises closer to the peak intensity, we can extract the reflectivity for different bunch densities, as shown in Fig. 1d . The strong increase in the intensity of the backscattered pulses due to the quadratic scaling on the electron density can clearly be seen in Fig. 1b . We can derive an expression for the coherent scattering from a dense electron bunch by extending the classical theory of Thomson scattering from a single electron to a system of N scatterers, taking into account the relative phase of each scattering electron. This problem is extensively discussed in the framework of scattering theory, or more specifically, in the theory of coherent synchrotron radiation [20] . Generally, the Thomson cross section of a single electron σ T =6.65 × 10 −25 cm 2 can be significantly enhanced in case of coherent scattering from a dense electron bunch with cross section σ coh = σ T | F | 2 , where F is the form factor of the electron bunch, that is the Fourier transform of the electron density. The electron bunches observed in PIC simulation can be modelled by a Gaussian profile and we find for the mirror reflectivity with . From simulation, we deduce that the REM thickness d is ~10 nm and can be regarded as rather constant for subsequent REMs. Assuming that in the transverse dimension electrons within the scattering section A = πλ r 2 contribute to the coherent signal [9] , we find a good agreement with the reflectivity extracted from PIC simulation, as shown in Fig. 1d . With the same values from above, the coherent enhancement of the reflected signal as compared with the incoherent scattering from N electrons is . How to cite this article: Kiefer D. et al . Relativistic electron mirrors from nanoscale foils for coherent frequency upshift to the extreme ultraviolet. Nat. Commun. 4:1763 doi: 10.1038/ncomms2775 (2013).